Quantum dot imaging platform for single-cell molecular profiling Study of normal cell physiology and disease pathogenesis heavily relies on untangling the complexity of intracellular molecular mechanisms and pathways. To achieve this goal, comprehensive molecular profiling of individual cells within the context of microenvironment is required. Here we report the development of a multicolour multicycle in situ imaging technology capable of creating detailed quantitative molecular profiles for individual cells at the resolution of optical imaging. A library of stoichiometric fluorescent probes is prepared by linking target-specific antibodies to a universal quantum dot-based platform via protein A in a quick and simple procedure. Surprisingly, despite the potential for multivalent binding between protein A and antibody and the intermediate affinity of this non-covalent bond, fully assembled probes do not aggregate or exchange antibodies, facilitating highly multiplexed parallel staining. This single-cell molecular profiling technology is expected to open new opportunities in systems biology, gene expression studies, signalling pathway analysis and molecular diagnostics. Comprehensive and quantitative molecular profiling on the single-cell level has the potential to unravel complex molecular pathways that underlie physiological and pathological processes, and thus represents a highly desirable tool for many applications that span the fields of systems biology, pathology, cell biology and clinical diagnostics [1] , [2] , [3] , [4] , [5] . The analytical power of such technologies comes from the synergistic use of two major strategies for cell characterization—single-cell measurements and multiplexed quantitative detection of molecular targets—that, when implemented separately, only provide partial insight on the state and behaviour of individual cells. For example, simultaneous analysis of multiple key molecular targets with multiplexed technologies, such as reverse-transcriptase PCR, gene chips, protein chips and mass spectrometry, is indispensable for describing the state of the cell population and its overall response to signalling, damage or therapeutic intervention. However, not only analysis of homogenized samples obscures unique states and responses of individual cells, but it also results in a loss of morphological information critical for evaluation of cell microenvironment [6] , [7] . On the other side, conventional staining methods, such as immunohistochemistry (IHC), are well-suited for examination of specimen morphology and assessing specimen heterogeneity through single-cell analysis, but often incapable to provide sufficient analytical and multiplexing capacity necessary for meaningful molecular profiling. Realizing the importance of comprehensive in situ single-cell molecular profiling, a number of advanced analytical techniques have been developed. For example, imaging mass spectrometry by far offers the greatest multiplexing capability, but it comes at a price of high equipment costs and much lower spatial resolution compared with optical imaging [8] , [9] . Mass cytometry, a technique utilizing lanthanides as highly multiplexable tags, offers single-cell quantitative analysis of antigen expression, but lacks imaging modality [10] , [11] , [12] . Surface-enhanced Raman scattering spectroscopy enables multiplexed molecular imaging, but suffers from the large surface-enhanced Raman scattering probe size (and, hence, limited specimen penetration) and slow pixel-by-pixel scanning process [13] , [14] , [15] , [16] . At the same time, numerous modifications have been proposed for improving analytical capabilities of conventional staining techniques. Building upon the conventional immunoenzyme staining, for example, modified protocols allow removal of chromogens post staining to restore samples for staining of a different set of targets [17] , [18] , [19] . Being highly laborious and time consuming, however, these improved IHC protocols are still limited to the detection of 3–4 antigens. In parallel, immunofluorescence (IF) by labelling antibodies with fluorophores has become an attractive alternative. Despite the broad availability of such probes, analysis is limited to qualitative evaluation of 2–3 colours in most cases owing to the unfavourable optical properties of organic dyes. Implementation of an automated cyclic IF has recently enabled interrogation of substantially larger sets of antigens using organic fluorophores [20] , [21] , [22] . However, numerous rounds of physical or chemical de-staining often lead to specimen degradation, whereas alternative approach of organic dye quenching through photobleaching hinders consistent quantitative signal analysis. In addition, interrogation of even a small number of molecular targets requires advanced instrumentation, making such technology inaccessible to most laboratories. In this context, major excitement took place with the introduction of semiconductor quantum dots (QDs) as fluorescent labels [23] , [24] and the recent advances in nanoparticle functionalization and bioconjugation [25] , [26] , [27] , [28] . These fluorescent nanocrystals exhibit unique optical properties, such as size-tunable and narrow emission spectra, simultaneous excitation of multiple colours, improved brightness and large Stokes shift, which are not available in either small molecules or bulk materials [3] , [29] . Furthermore, in contrast to organic fluorophores, QDs demonstrate outstanding photostability ( Supplementary Fig. S1 ) that enables consistent image acquisition critical for accurate quantitative signal analysis. As a result, QDs are uniquely suited for highly multiplexed quantitative molecular profiling in a conventional laboratory setting, requiring minimal instrumentation changes (such as use of narrow band-pass filters or hyperspectral imaging (HSI) camera [30] ). For example, simultaneous detection of at least ten different colours within the spectral range (400–900 nm) of common charge-coupled devices is currently achievable. Despite this promise, QD-based fluorescence imaging has yet to show major improvements over organic dyes, as current multiplexing capability is far below the expectation of creating a truly comprehensive molecular portrait for individual cells (the state of the art is imaging of 5–6 molecular targets with custom-designed QD probes) [31] , [32] , [33] , [34] , [35] . To fully utilize the extensive multiplexing potential of QDs and take advantage of the wide selection of validated primary antibodies for molecular profiling with IF, here, we report the development of a multicolour multicycle molecular profiling (M3P) technology potentially capable of examining over 100 molecular targets in single cells at subcellular resolution. We achieve this goal by first engineering a universal QD-protein A (QD-SpA) platform for flexible and fast preparation of a library of functional QD-antibody (QD-SpA-Ab) probes and utilizing such probes in a multicycle staining procedure. To demonstrate the concept and feasibility, in this paper we show that at least 25 targets (5 colours × 5 cycles) can be reliably imaged with subcellular resolution and analysed quantitatively, while also attesting that M3P technology can be expanded to evaluation of 50–100 targets in a straightforward manner. Featuring a unique combination of quantitative multiplexed analysis and HSI-aided high-resolution fluorescence microscopy, the M3P platform described here should enable extensive single-cell molecular profiling studies on specimens with preserved morphology, a task unachievable by current state-of-the-art techniques. M3P platform design Unique optical properties of QD probes in combination with expanded multiplexing capacity of cyclic staining methodology offer straightforward and robust route to quantitative examination of single-cell molecular profiles. However, implementation of a QD-based multicolour multicycle technology heavily depends on addressing several key challenges: (i) each QD probe must be uniquely matched to a specific target, exhibiting no crosstalk between different probes within a staining cocktail; (ii) QD fluorescence must be completely removed after each imaging cycle to prevent signal carry-over to the next staining cycle; and (iii) target antigenicity and specimen integrity must be retained throughout multiple staining/imaging/de-staining cycles. In addition, practical considerations associated with these conditions should be met. In particular, current lack of flexible, simple and cost-effective route for QD-Ab probe preparation represents a major roadblock on the way towards implementation of molecular profiling concept, as inefficient and expensive chemical conjugation between 1′Abs and QDs (some commercially available as kits) [35] , [36] severely limits the use of QD technology to only a few proof-of-concept studies performed by specialized laboratories. The M3P technology described here has been designed to completely address demanding conditions for comprehensive in situ cell profiling. A universal nanoparticle platform, QD-SpA, has been engineered for on-demand single-step purification-free preparation of QD-SpA-Ab probes via non-covalent self-assembly, thus significantly lowering cost, streamlining assay development and making this method accessible to a wide range of biomedical researchers. At the same time, specimen regeneration methodology taking advantage of the semi-stable nature of the SpA–Ab interaction has been developed for ready probe elution and unhampered target labelling through multiple cycles. As schematically illustrated in Fig. 1 , the M3P technology consists of three main steps. First, universal QD–SpA bioconjugates are used to capture intact Abs in solution during a pre-staining step to form functional QD-SpA-Ab fluorescent probes ( Fig. 1a ). Once formed, different probes are pooled in a single cocktail ( Fig. 1b ) and incubated with cells for parallel multiplexed staining ( Fig. 1c ). In the second step, fluorescence microscopy with HSI capability [32] is utilized to acquire and unmix signals from each QD colour to generate quantitative antigen expression profiles in separate channels ( Fig. 1d ). In the third step, complete de-staining of the specimen is done by brief washing with a regeneration buffer ( Fig. 1e ), enabling the next full cycle of IF staining for a different subset of targets ( Fig. 1f ). With each staining cycle, N targets can be analysed, where N depends on the number of spectrally distinct fluorescent probes that can be detected simultaneously. Performing IF staining for M sequential cycles generates M subsets of data for the same specimen, thus yielding an overall molecular profile consisting of N × M targets. For example, ten spectrally distinct QDs with at least 20 nm separation between fluorescence maxima are commercially available currently and can be linked to ten Abs. This multiplexing capability is complemented by the spectral unmixing power of HSI (also ten channels at this time) for separation and quantification of individual colours from multicolour images. When the staining/imaging procedure is carried out for ten cycles, 10 × 10 (100) molecular targets can be studied within a single sample. 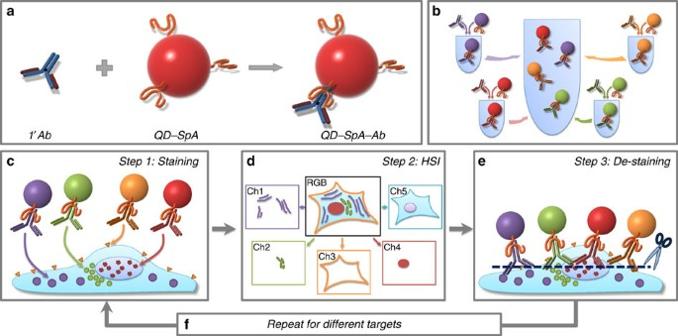Figure 1: Schematic illustration of the M3P technology. (a) A universal QD-SpA platform is used for single-step purification-free assembly of functional QD-SpA-Ab probes via capture of free antibodies from solution by SpA. (b) Once bound, Abs cannot be exchanged between QD-SpA probes, thus enabling mixing of multicolour probes within a single cocktail. (c) The QD-SpA-Ab cocktail is used for single-step parallel multiplexed staining. (d) Spectral imaging is performed for unmixing individual QD colours, quantitative analysis of target expression and depiction of relative target distribution within the specimen. (e) Complete de-staining restores specimen for another staining cycle. (f) Sequential repetition ofN-colour parallel staining forMcycles enables analysis ofN×Mmolecular targets. Figure 1: Schematic illustration of the M3P technology. ( a ) A universal QD-SpA platform is used for single-step purification-free assembly of functional QD-SpA-Ab probes via capture of free antibodies from solution by SpA. ( b ) Once bound, Abs cannot be exchanged between QD-SpA probes, thus enabling mixing of multicolour probes within a single cocktail. ( c ) The QD-SpA-Ab cocktail is used for single-step parallel multiplexed staining. ( d ) Spectral imaging is performed for unmixing individual QD colours, quantitative analysis of target expression and depiction of relative target distribution within the specimen. ( e ) Complete de-staining restores specimen for another staining cycle. ( f ) Sequential repetition of N -colour parallel staining for M cycles enables analysis of N × M molecular targets. Full size image QD-Ab probe preparation In contrast to dye molecules, ultrasensitive detection and imaging with nanoparticle-based probes require complete neutralization of particle surface charge for suppression of nonspecific staining [3] , [25] , [37] . Therefore, as a platform for M3P technology, we use highly stable and bright QDs coated with a non-fouling layer of polyethylene glycol (PEG). With proper specimen blocking, these particles produce no detectable nonspecific specimen staining. Protein A from Staphylococcus aureus (SpA) is covalently linked to QDs as an adaptor for orientation-controlled IgG immobilization via binding to the Fc region of IgG. Such selective SpA-mediated IgG capture and lack of other interactions between specimen and non-functionalized QD-SpA probes ensure highly specific staining in a stoichiometric manner ( Supplementary Fig. S2 ). Other adaptor proteins, such as protein G and streptavidin, may be used in a similar fashion, but it must be assured that there are no sterically accessible binding sites left on Ab after QD–Ab complex formation to prevent crosslinking of different QDs via Abs. In this regard, SpA possesses five IgG-binding sites [38] , two of which are accessible simultaneously, while IgG has two SpA-binding sites on its Fc region, making formation of polymeric SpA–IgG complexes possible [39] , [40] , [41] , [42] . To our surprise, however, no aggregation was observed between QD-SpA and IgG by fluorescence microscopy and dynamic light scattering. We attribute this effect to potential divalent binding of both sites on IgG by SpA attached to QD surface, which is favoured when the molar ratio of SpA to IgG is relatively high [41] . Furthermore, covalent attachment of SpA to nanoparticle surface hampers formation of the aforementioned SpA-IgG oligomer structure owing to steric hindrance, thus offering an additional mechanism in preventing probe crosslinking. Performance of the QD-SpA-Ab probes is qualitatively assessed by staining five molecular targets separately in formalin-fixed HeLa cells ( Fig. 2a ) and comparing the relative target distribution patterns with those obtained by conventional two-step IF using commercially available QD-labelled 2′Ab ( Fig. 2b ) and Alexa Fluor 568-labelled 2′Ab ( Fig. 2c ). The five model targets used in this study (Ki-67, HSP90, Lamin A, Cox-4 and β-tubulin) represent a spectrum of cell compartment localizations and expression levels. Remarkably, the staining patterns are consistent throughout all three procedures, indicating preserved specificity and affinity of antibodies in the QD–SpA–Ab complex. 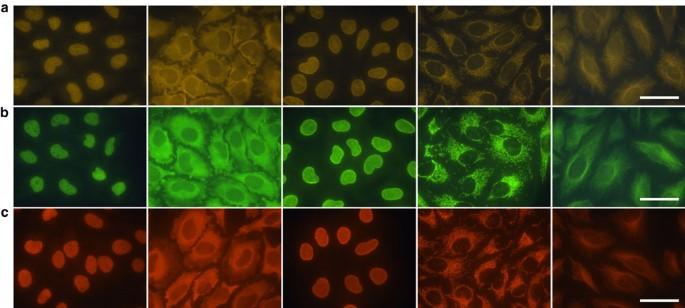Figure 2: Characterization of QD-Ab probe specificity. (a) Five model targets (Ki-67, HSP90, Lamin A, Cox-4 and β-tubulin, from left to right) are labelled with QD585-SpA-Ab probes in a single-step procedure, producing staining patterns consistent with those obtained with either QD565-labelled (b) or Alexa Fluor 568-labelled (c) 2′Abs in a conventional two-step staining. Scale bar, 50 μm. Figure 2: Characterization of QD-Ab probe specificity. ( a ) Five model targets (Ki-67, HSP90, Lamin A, Cox-4 and β-tubulin, from left to right) are labelled with QD585-SpA-Ab probes in a single-step procedure, producing staining patterns consistent with those obtained with either QD565-labelled ( b ) or Alexa Fluor 568-labelled ( c ) 2′Abs in a conventional two-step staining. Scale bar, 50 μm. Full size image Quantitative evaluation of staining with QD-SpA-Ab probes is done through staining of three of the five model targets (Lamin A for nuclear membrane, HSP90 for cytoplasm and Cox-4 for mitochondria) with all QD colours and using HSI for image acquisition and signal analysis. First, utility of HSI for spectral unmixing of QD probes is confirmed ( Supplementary Fig. S3a ) and differential brightness of different QD probes is assessed ( Supplementary Fig. S3b ) through HSI analysis of bulk QD solutions. Then, relative staining intensity obtained with five QD colours is compared between the three targets probed and with bulk fluorescence measurements ( Supplementary Fig. S3c ). Consistency of observed differential QD brightness throughout staining experiments and bulk measurements indicates unhampered access of all QD-SpA-Ab probes to intracellular targets and corroborates robustness of HSI-based quantitative analysis of staining intensity. Consistent kinetics of target staining with different QD probes, essential for achieving the same degree of labelling regardless of the QD probe used, is verified for QDs emitting at 525 and 605 nm, which represent nanocrystals with smallest and largest inorganic cores, respectively ( Supplementary Fig. S4 ). Despite the differences in core size, both probes demonstrate identical time evolution of HSP90 staining intensity, reaching a plateau after about 2 h of incubation ( Supplementary Fig. S4a,b ). This behaviour is perhaps not surprising, as the differences in core size are equalized to a great extent by the thick organic coating layers, as is the case with QD-SpA probes used here ( Supplementary Fig. S4c ). QD-SpA-Ab probe stability for multicolour staining For practical application of the M3P technology, linking functional QD probes with Abs of interest should be quick and simple, as opposed to conventional techniques relying on complex chemical reactions and purifications for each Ab [28] , [35] . The assembly of QD–Ab bioconjugates in our technology is done by simple mixing of QD-SpA and primary Ab. SpA binds a wide range of antibodies with an intermediate affinity (Kd on the order of 10 −8 –10 −10 M). Therefore, by incubating QD–SpA complexes in excess to antibodies before staining, nearly complete capture of antibodies by QD-SpA is expected, thus preventing binding of free IgG to vacant SpA sites on different QD-SpA probes. However, considering that all QD-SpA-Ab probes form via the same non-covalent SpA–Ab bond, spontaneous QD–SpA–Ab dissociation, Ab exchange and crosstalk between different probes (that is, labelling of a wrong target by QD-SpA probe owing to capture of free or specimen-bound IgG during staining procedure) cannot be completely ruled out. To probe this critical issue, we studied the SpA–Ab dissociation kinetics using SPR (surface plasmon resonance)-based real-time analysis and assessed QD-SpA-Ab probe stability and potential for crosstalk experimentally with dual-colour staining. For SPR studies, SpA is immobilized on dextran-coated chip, and binding of excess rabbit anti-mouse IgG to immobilized SpA in reference to control unmodified surface is recorded. We observe overall lower binding affinity when analyte is injected at high concentration (250 nM–4 μM) with a K d up to 100 times higher than that for low-concentration analyte (10 nM–250 nM). Measurements of binding and dissociation kinetics show a nonlinear behaviour, which is especially pronounced for the high-concentration analyte. This observation is consistent with early reports suggesting that slow binding and dissociation by strong binding sites is accompanied with fast binding and dissociation via weak sites, especially when strong sites are saturated [43] . In light of the proposed divalent SpA-Ab-binding model, we hypothesize that strong binding with slow kinetics might occur owing to capture of both IgG-binding sites by two different subunits of the same SpA (which is favoured under non-saturating conditions) [40] , [41] or two neighbour surface-bound SpA molecules, while monovalent SpA-IgG binding results in weak and fast interaction (under saturating conditions). Indeed, in the relatively low concentration range, the dissociation curve for 100 nM Ab shows an initial fast drop in signal, accounting for about 5% loss of bound Ab, followed by a very slow dissociation ( Supplementary Fig. S5a ). The same measurements performed with 10 nM Ab, which is consistent with the final Ab concentration used in the staining experiments, show nearly no SpA–Ab dissociation for 60 min ( Supplementary Fig. S5b ). These results suggest that the SpA–Ab dissociation kinetics is sufficiently slow at the concentration range and time frame of the cell staining procedure to prevent QD–SpA–Ab complex disassembly and release of free antibodies in solution. However, it is critical to ensure that excess of QD-SpA probes over Abs is used in the initial mixing step to favour formation of stable SpA–Ab bonds and avoid QD-SpA surface saturation. To further test the QD-SpA-Ab stability and directly answer the question whether crosstalk exists in multicolour cell staining, we prepared two QD-SpA-Ab probes emitting at 545 and 585 nm. We chose Lamin A as the staining target for its high expression in HeLa cells and the distinct nuclear envelope localization. Immediately before staining, we mixed fully assembled QD-SpA-Ab probes with counterpart non-complexed QD-SpA (for example, QD545-SpA-Ab mixed with QD585-SpA, or QD585-SpA-Ab with QD545-SpA), and incubated cells with this solution. If crosstalk exists, with this setup, the large excess of vacant counterpart QD-SpA probes would bind any free Ab released from the QD-SpA-Ab probes and compete for target binding. Remarkably, we did not observe any crosstalk or interference with either QD545 or QD585 probes ( Fig. 3b–e ). At the same time, QD545-SpA and QD585-SpA probes mixed together with Ab and incubated with cells efficiently captured free Ab from solution and produced mixed-colour Lamin A staining with nearly 50% contribution each ( Fig. 3a ). From these two independent measurements (SPR analysis and cell staining), we conclude that pre-assembled QD–SpA–Ab complexes, featuring very slow dissociation kinetics and sterically blocked access to bound Abs, do not exchange Abs with other vacant QD-SpA probes within the concentration range and time frame of the cell staining experiment. In addition, slow diffusion of the relatively large QD–SpA bioconjugates might further reduce capacity for recapture of rare free IgG that might be spontaneously released by the QD-SpA-Ab probes. This cornerstone property of QD-SpA probes forms the foundation for reliable and specific parallel multiplexed staining. 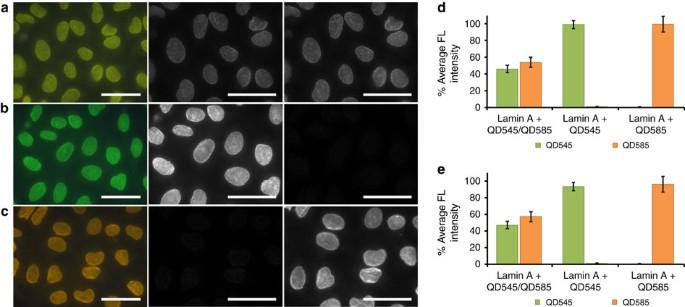Figure 3: Characterization of QD-SpA-Ab probe stability. (a) As QD-SpA can capture free Abs from solution, when anti-Lamin A IgG, QD545-SpA and QD585-SpA are mixed simultaneously and immediately applied to cells, both probes successfully capture Ab and produce Lamin A staining with ~50% contribution from each (a,d). At the same time, regardless of whether QD545 (b) or QD585 (c) is pre-assembled with anti-Lamin A antibody, only the pre-assembled probe shows specific nuclear envelope staining, solely contributing to all fluorescence signal registered (d). Furthermore, presence of a competitor QD-SpA probe does not interfere with target staining by the pre-assembled QD-SpA-Ab probe, as observed signal intensity in a two-probe mixture is comparable to that obtained with single-colour staining experiments in the absence of a competitor probe (e). HSI is used to unmix true-colour images (left panels) into individual QD545 (middle panels) and QD585 (right panels) channels, remove background and perform quantitative analysis of staining intensity. Brightness of individual QD channels is normalized to aid in direct comparison of staining intensity. Intensity of the QD545 channel is scaled up by a factor of 2 relative to QD585 channel to compensate for differential brightness of QD probes. Error bars represent s.d. of the average staining intensity between three different fields of view imaged on the same specimen. FL intensity denotes fluorescence QD signal intensity measured by HSI. Scale bar, 50 μm. Figure 3: Characterization of QD-SpA-Ab probe stability. ( a ) As QD-SpA can capture free Abs from solution, when anti-Lamin A IgG, QD545-SpA and QD585-SpA are mixed simultaneously and immediately applied to cells, both probes successfully capture Ab and produce Lamin A staining with ~50% contribution from each ( a , d ). At the same time, regardless of whether QD545 ( b ) or QD585 ( c ) is pre-assembled with anti-Lamin A antibody, only the pre-assembled probe shows specific nuclear envelope staining, solely contributing to all fluorescence signal registered ( d ). Furthermore, presence of a competitor QD-SpA probe does not interfere with target staining by the pre-assembled QD-SpA-Ab probe, as observed signal intensity in a two-probe mixture is comparable to that obtained with single-colour staining experiments in the absence of a competitor probe ( e ). HSI is used to unmix true-colour images (left panels) into individual QD545 (middle panels) and QD585 (right panels) channels, remove background and perform quantitative analysis of staining intensity. Brightness of individual QD channels is normalized to aid in direct comparison of staining intensity. Intensity of the QD545 channel is scaled up by a factor of 2 relative to QD585 channel to compensate for differential brightness of QD probes. Error bars represent s.d. of the average staining intensity between three different fields of view imaged on the same specimen. FL intensity denotes fluorescence QD signal intensity measured by HSI. Scale bar, 50 μm. Full size image To demonstrate the utility of the new probes for multicolour imaging, parallel staining of five model molecular targets is performed. Similar to the single-colour staining discussed above, individual QD-SpA probes and corresponding Abs are first incubated for 1 h separately, and then pooled together for staining. HSI reveals that the QD–SpA–Ab bioconjugates can reliably detect intracellular distribution ( Fig. 4a–c ) and relative expression levels ( Fig. 4d ) of different targets regardless of their cellular location. Furthermore, identical relative target expression profiles are obtained with multiplexed, singleplexed multicolour and singleplexed single-colour staining ( Fig. 4d ), confirming robustness of quantitative signal analysis in a multiplexed format. It is also worth emphasizing once again that in this multicolour unmixing process, the remarkable brightness and photostability of QDs enables reliable image acquisition by scanning through a broad spectral range with narrow bandwidth, while less stable organic fluorophores would rapidly quench during imaging. 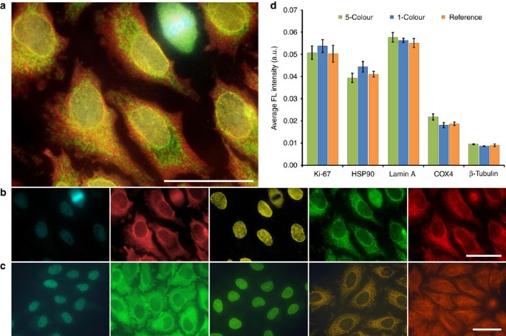Figure 4: Parallel multiplexed staining with five pre-assembled QD-SpA-Ab probes. Ki-67, HSP90, Lamin A, Cox-4 and β-tubulin are simultaneously stained with QD-SpA-Ab probes emitting at 525, 545, 565, 585 and 605 nm, respectively (a). HSI and spectral unmixing are used to extract individual QD channels (b), perform quantitative analysis of staining intensity (d) and reconstruct a false-colour composite image (a) depicting relative distribution and colocalization of different targets. Staining patterns obtained in this manner (b) are consistent with single-colour staining performed with colour-matched QD-SpA-Ab probes (c). Furthermore, average staining intensities for five model targets measured with multiplexed staining (five-colour bars ind) are consistent with quantitative analysis performed with singleplexed staining using either colour-matched QD-SpA-Ab probes (single-colour bars ind) or reference singleplexed staining performed with same QD585-SpA probe for all targets (reference bars ind). Individual channels (b) are false-coloured and fluorescence intensity of individual channels is automatically adjusted by HSI software to achieve clear target representation in a composite false-colour image (a). For quantitative analysis (d), fluorescence intensity of individual QDs is normalized to reference QD585 using appropriate correction factor (Supplementary Fig. S3). Error bars represent s.d. of the average staining intensity between three different fields of view imaged on the same specimen. FL intensity denotes fluorescence QD signal intensity measured by HSI. Scale bar, 50 μm. Figure 4: Parallel multiplexed staining with five pre-assembled QD-SpA-Ab probes. Ki-67, HSP90, Lamin A, Cox-4 and β-tubulin are simultaneously stained with QD-SpA-Ab probes emitting at 525, 545, 565, 585 and 605 nm, respectively ( a ). HSI and spectral unmixing are used to extract individual QD channels ( b ), perform quantitative analysis of staining intensity ( d ) and reconstruct a false-colour composite image ( a ) depicting relative distribution and colocalization of different targets. Staining patterns obtained in this manner ( b ) are consistent with single-colour staining performed with colour-matched QD-SpA-Ab probes ( c ). Furthermore, average staining intensities for five model targets measured with multiplexed staining (five-colour bars in d ) are consistent with quantitative analysis performed with singleplexed staining using either colour-matched QD-SpA-Ab probes (single-colour bars in d ) or reference singleplexed staining performed with same QD585-SpA probe for all targets (reference bars in d ). Individual channels ( b ) are false-coloured and fluorescence intensity of individual channels is automatically adjusted by HSI software to achieve clear target representation in a composite false-colour image ( a ). For quantitative analysis ( d ), fluorescence intensity of individual QDs is normalized to reference QD585 using appropriate correction factor ( Supplementary Fig. S3 ). Error bars represent s.d. of the average staining intensity between three different fields of view imaged on the same specimen. FL intensity denotes fluorescence QD signal intensity measured by HSI. Scale bar, 50 μm. Full size image Multicycle imaging with QD-SpA-Ab probes M3P technology enables expansion of the multiplexing capability of QD-based IF by another magnitude through a sequential cyclic staining procedure. Microwave treatment [19] , strong acidic conditions [17] , [18] , [20] and specimen dehydration [17] have been used with some success for sequential staining procedures based on conventional IF and IHC. However, elimination of large staining complexes (often consisting of crosslinked primary and secondary Abs conjugated with enzymes or streptavidin and surrounded by precipitated chromogens) proves to be challenging and requires extensive chemical or thermal treatment, which could lead to specimen degradation. With the new QD-SpA-Ab probes, directly benefiting from the non-covalent semi-stable nature of the probe assembly, we achieve quick and efficient de-staining by brief exposure to low-pH/detergent-based regeneration buffer, because (i) the staining procedure does not involve formation of large precipitates; (ii) antigen–Ab and SpA–Ab bonds can be easily broken by exposure to low pH and detergent; and (iii) trace amount of residual QDs, if any, is completely quenched. To test this technique, Lamin A is stained with QD605 ( Supplementary Fig. S6a ) and de-stained by incubation with regeneration buffer, leaving no leftover QD605 signal ( Supplementary Fig. S6b ). Secondary detection of QD605-SpA probes through SpA staining with QD565 reveals that nearly all (>90%) QD-SpA probes are eluted from the specimen during de-staining ( Supplementary Fig. S6d,e ). At the same time, when QD605-SpA-Ab probes are covalently crosslinked to cells, all probes remain bound to their targets, but produce no fluorescence signal owing to irreversible quenching of QD fluorescence ( Supplementary Fig. S6c,f ). Taken together, these results show that de-staining is achieved primarily by dissociation of QD-SpA-Ab probes from the specimen and completed by quenching of leftover QDs, thus restoring the specimen to pre-staining condition. Notably, specimen regeneration through QD-SpA-Ab probe elution releases targets of their labels, thus enabling complete re-staining of the same targets during subsequent cycles. For example, Lamin A stained with QD545 can be re-stained again with pre-assembled QD545-SpA-Ab probe, while ‘blank’ QD545-SpA fails to produce any staining ( Fig. 5a–d ). Similarly, in a dual-colour staining of Lamin A and HSP90 with QD545 and QD585 probes, respectively ( Fig. 5e–h ), we achieve complete exchange of fluorescent reporters during the second cycle ( Fig. 5i–l ) and measure identical relative average staining intensities for these targets during both cycles. While re-staining of targets might be unnecessary in majority of cell profiling applications, complete removal of QD-SpA-Ab probes is still desirable to avoid any steric hindrance that may be encountered by nanoprobes during cyclic staining of closely spaced targets. Therefore, given restaining results, it is reasonable to conclude that such an issue should not arise with M3P technology. 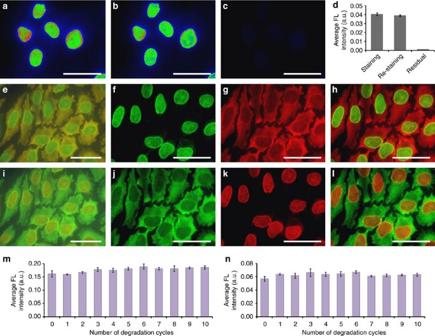Figure 5: Specimen regeneration and target re-staining with multicycle staining procedure. (a) Characteristic nuclear envelope staining is obtained with QD545-SpA probes pre-assembled with anti-Lamin A antibody. Brief incubation with regeneration buffer removes QD-SpA-Ab probes, achieving specimen restoration to pre-staining condition and enabling nearly complete target re-staining (b,d). At the same time, incubation of regenerated specimen with ‘blank’ QD545-SpA probes (lacking target-specific Abs) fails to produce any residual staining (c,d), confirming complete removal of 1'Abs during de-staining. Same subset of cells is imaged, normalized by intensity and false-coloured with a heat map for this study. (e–l) Further application of the de-staining/re-staining procedure to dual-colour cell labelling enables complete exchange of QD reporters between two different molecular targets. Specifically parallel staining of Lamin A with QD545 and HSP90 with QD585 is achieved (e–h). HSI reveals distinct Lamin A staining pattern in QD545 channel (f) and HSP90 pattern in QD585 channel (g). Following de-staining, during the second cycle the same targets are stained with the counterpart QD probes (i–l), yielding clear HSP90 pattern in QD545 channel (j) and Lamin A pattern in QD585 channel (k). (e) and (i) are true-colour images and (h) and (l) are false-colour composite images. Fluorescence intensity of individual channels is adjusted to achieve clear target representation in composite false-colour images. Same subpopulation of cells is imaged after each step to aid in direct comparison of staining patterns. To quantitatively assess effect of repeated regeneration procedure on specimen stability and staining intensity, up to 10 ‘degradation’ cycles are performed on separate specimens before cells are stained for Lamin A (m) or HSP90 (n). For both targets, measured average fluorescence staining intensity does not vary significantly regardless of the number of ‘degradation’ cycles performed, demonstrating sufficient preservation of specimen antigenicity required for cyclic staining. Error bars represent s.d. of the average staining intensity between four different fields of view imaged on the same specimen. FL intensity denotes fluorescence QD signal intensity measured by HSI. Scale bar, 50 μm. Figure 5: Specimen regeneration and target re-staining with multicycle staining procedure. ( a ) Characteristic nuclear envelope staining is obtained with QD545-SpA probes pre-assembled with anti-Lamin A antibody. Brief incubation with regeneration buffer removes QD-SpA-Ab probes, achieving specimen restoration to pre-staining condition and enabling nearly complete target re-staining ( b , d ). At the same time, incubation of regenerated specimen with ‘blank’ QD545-SpA probes (lacking target-specific Abs) fails to produce any residual staining ( c , d ), confirming complete removal of 1'Abs during de-staining. Same subset of cells is imaged, normalized by intensity and false-coloured with a heat map for this study. ( e – l ) Further application of the de-staining/re-staining procedure to dual-colour cell labelling enables complete exchange of QD reporters between two different molecular targets. Specifically parallel staining of Lamin A with QD545 and HSP90 with QD585 is achieved ( e – h ). HSI reveals distinct Lamin A staining pattern in QD545 channel ( f ) and HSP90 pattern in QD585 channel ( g ). Following de-staining, during the second cycle the same targets are stained with the counterpart QD probes ( i – l ), yielding clear HSP90 pattern in QD545 channel ( j ) and Lamin A pattern in QD585 channel ( k ). ( e ) and ( i ) are true-colour images and ( h ) and ( l ) are false-colour composite images. Fluorescence intensity of individual channels is adjusted to achieve clear target representation in composite false-colour images. Same subpopulation of cells is imaged after each step to aid in direct comparison of staining patterns. To quantitatively assess effect of repeated regeneration procedure on specimen stability and staining intensity, up to 10 ‘degradation’ cycles are performed on separate specimens before cells are stained for Lamin A ( m ) or HSP90 ( n ). For both targets, measured average fluorescence staining intensity does not vary significantly regardless of the number of ‘degradation’ cycles performed, demonstrating sufficient preservation of specimen antigenicity required for cyclic staining. Error bars represent s.d. of the average staining intensity between four different fields of view imaged on the same specimen. FL intensity denotes fluorescence QD signal intensity measured by HSI. Scale bar, 50 μm. Full size image Expansion of M3P technology to profiling of over 100 molecular targets, nonetheless, requires that at least ten cycles of staining are performed (assuming parallel use of ten QD colours complemented by 10-channel HSI), thus placing restrictions on regeneration conditions. Acknowledging this requirement, we have verified that with optimized procedure used here up to (but not limited to) ten regeneration cycles can be performed with no detrimental effect on specimen morphology and target antigenicity (as tested with Lamin A, Fig. 5m , and HSP90, Fig. 5n ). Specifically, we designed experiments using cells located in separate wells of the same 24-well plate, thus ensuring that all cells were prepared under identical conditions. Cells were exposed to M regeneration cycles (where M ranged from 0–10). Each cycle consisted of de-staining, blocking, incubation with staining buffer and washing, imitating a full IF staining cycle. Following the multicycle treatment, Lamin A and HSP90 were stained, and HSI was used for quantitative analysis of average staining intensities. Consistent staining observed regardless of the number of regeneration cycles performed supports further expansion of the multicycle staining with M3P technology. Complete specimen regeneration paired with lack of specimen degradation enables robust singleplex cyclic staining of the five model molecular targets regardless of the target expression levels and staining sequence ( Fig. 6 ). For example, we show here that correct staining pattern and target expression profile can be obtained for staining sequence from highly condensed Lamin A down to diffusely distributed β-tubulin ( Fig. 6a–c ) and in reverse ( Fig. 6d–f ), both matching relative profile obtained from reference singleplex single-cycle staining with QD585-SpA ( Fig. 6g ). Attesting to efficiency of de-staining procedure, no carry-over or residual staining is detectable throughout the five cycles. 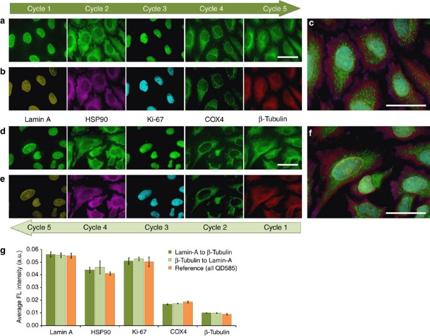Figure 6: Evaluation of the robustness of sequential staining procedure. Single-colour staining of five molecular targets (Lamin A, HSP90, Ki-67, Cox-4 and β-tubulin) on the same cell subpopulation is performed using QD545-SpA-Ab probes in sequential manner in the order from highly condensed to diffusely distributed targets (Lamin A to β-tubulin,a–c) and in reverse (β-tubulin to Lamin A,d–f). Quantitative analysis of target staining intensity for both sequences in comparison with reference single-cycle single-colour staining performed with QD585-SpA probes is shown in (g). Independent of the order, all targets are reliably stained, showing correct staining pattern and relative staining intensity. No carry-over fluorescence, build-up of background fluorescence or cross-staining between cycles can be observed. Original images obtained with HSI (a,d) are false-coloured, aligned and cropped (b,e) for clear representation of each target in composite false-colour images (c,f). Error bars represent s.d. of the average staining intensity between three different fields of view imaged on the same specimen. FL intensity denotes fluorescence QD signal intensity measured by HSI. Scale bar, 50 μm. Figure 6: Evaluation of the robustness of sequential staining procedure. Single-colour staining of five molecular targets (Lamin A, HSP90, Ki-67, Cox-4 and β-tubulin) on the same cell subpopulation is performed using QD545-SpA-Ab probes in sequential manner in the order from highly condensed to diffusely distributed targets (Lamin A to β-tubulin, a – c ) and in reverse (β-tubulin to Lamin A, d – f ). Quantitative analysis of target staining intensity for both sequences in comparison with reference single-cycle single-colour staining performed with QD585-SpA probes is shown in ( g ). Independent of the order, all targets are reliably stained, showing correct staining pattern and relative staining intensity. No carry-over fluorescence, build-up of background fluorescence or cross-staining between cycles can be observed. Original images obtained with HSI ( a , d ) are false-coloured, aligned and cropped ( b , e ) for clear representation of each target in composite false-colour images ( c , f ). Error bars represent s.d. of the average staining intensity between three different fields of view imaged on the same specimen. FL intensity denotes fluorescence QD signal intensity measured by HSI. Scale bar, 50 μm. Full size image Implementation of M3P technology for 25-target profiling Comprehensive single-cell molecular profiling with M3P technology is implemented by joining multicolour and multicycle staining modalities described above. Parallel multicolour staining features capacity for simultaneous analysis of up to ten targets, whereas sequential single-colour staining also enables robust interrogation of at least ten (or more) targets through several cycles. Therefore, when combined together, these modalities potentially offer access to quantitative molecular profiles consisting of 100+ molecular targets. We demonstrate the feasibility or such an extensive molecular profiling capacity by performing a 25-target analysis in a 5-colour × 5-cycle format. Specifically, we re-stain the same model 5-target panel (Ki-67, HSP90, Lamin A, Cox-4 and β-tubulin) with multicolour QD-SpA-Ab probes for five cycles and perform quantitative analysis of staining intensity after each cycle. Such setup facilitates not only the demonstration of the concept, but also further evaluation of the technology robustness, including assessment of the target staining pattern consistency, preservation of subcellular and cell culture morphology, and uniformity of relative target expression profiles measured through different staining cycles. Notably, all five targets are consistently stained through five cycles yielding accurate staining patterns and identical average staining intensity profiles ( Fig. 7 ), while producing no carry-over of fluorescence signal between cycles ( Supplementary Fig. S7 ). Furthermore, low-magnification imaging of the same field of view demonstrates complete preservation of cell culture morphology through five cycles ( Supplementary Fig. S8 ). 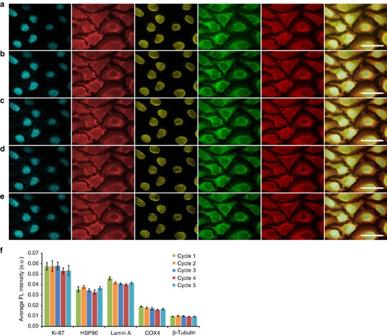Figure 7: Validation of M3P technology with 25-target staining. Utility of M3P technology for highly multiplexed molecular profiling is demonstrated by re-staining the same set of five model molecular targets (Ki-67, HSP90, Lamin A, Cox-4 and β-tubulin labelled with QD-SpA-Ab probes emitting at 525, 545, 565, 585 and 605 nm, respectively) through five cycles (a–e) and performing quantitative analysis of average staining intensity for each target at every cycle (f). Qualitative evaluation of individual QD channels (columns 1–5 ina–e) as well as composite images (column 6 ina–e) of the same cell subpopulation imaged after every cycle shows robust re-staining of each target with precisely preserved subcellular morphology, whereas quantitative analysis (f) demonstrates consistency of target staining profiles throughout all cycles. Note that complete specimen regeneration is achieved after each cycle, leaving no detectable fluorescence signal (Supplementary Fig. S7), thus ensuring that observed staining is generated by incubation of cells with a new QD-SpA-Ab cocktail during each cycle. Error bars represent s.d. of the average staining intensity between three different fields of view imaged on the same specimen. FL intensity denotes fluorescence QD signal intensity measured by HSI. Scale bar, 50 μm. Figure 7: Validation of M3P technology with 25-target staining. Utility of M3P technology for highly multiplexed molecular profiling is demonstrated by re-staining the same set of five model molecular targets (Ki-67, HSP90, Lamin A, Cox-4 and β-tubulin labelled with QD-SpA-Ab probes emitting at 525, 545, 565, 585 and 605 nm, respectively) through five cycles ( a – e ) and performing quantitative analysis of average staining intensity for each target at every cycle ( f ). Qualitative evaluation of individual QD channels (columns 1–5 in a – e ) as well as composite images (column 6 in a – e ) of the same cell subpopulation imaged after every cycle shows robust re-staining of each target with precisely preserved subcellular morphology, whereas quantitative analysis ( f ) demonstrates consistency of target staining profiles throughout all cycles. Note that complete specimen regeneration is achieved after each cycle, leaving no detectable fluorescence signal ( Supplementary Fig. S7 ), thus ensuring that observed staining is generated by incubation of cells with a new QD-SpA-Ab cocktail during each cycle. Error bars represent s.d. of the average staining intensity between three different fields of view imaged on the same specimen. FL intensity denotes fluorescence QD signal intensity measured by HSI. Scale bar, 50 μm. Full size image QD-based probes have become an indispensable tool for quantitative multiplexed studies, enabling simultaneous detection and analysis of multiple targets within a single specimen. Importantly, outstanding QD photostability proves essential for robust image acquisition and accurate quantitative analysis of staining intensity, which is a fundamental limitation of organic fluorophore-based methods. Advances in QD synthesis and surface modification achieved during the last decade have produced multicolour QD–Ab bioconjugates aiming to expand multiplexing capabilities of IF staining. However, truly multiplexed and quantitative molecular profiling of single cells and clinical tissue specimens remains elusive. Common two-step IF staining based on consecutive labelling with 1′Ab and 2′Ab-QD (or 1′Ab-biotin and QD-streptavidin) is strictly limited by the lack of suitable 1′Ab/2′Ab pairs or by the biotin–streptavidin interaction, thus demonstrating only modest multiplexing [31] , [44] , [45] . This limitation can be resolved to some extent by performing the two-step staining procedure on the same specimen multiple times in sequential manner [33] , [34] , but owing to the multivalency of QD probes, crosstalk between different staining cycles is virtually inevitable as newly introduced 1′Abs necessarily bind to unoccupied sites of QD-2′Ab from previous rounds. Single-step staining has also been achieved by covalent linking of QDs to 1′Abs (which requires Abs free of carrier proteins), thus eliminating the 1′Ab/2′Ab species limitation [35] . However, chemical modification and purification steps involved in the direct conjugation process are not only highly complex and prohibitively expensive but also often result in reduction in antibody avidity. To accommodate the needs and requirements of a wide range of biomedical applications, M3P of single cells and tissue specimens must be based on production of QD-Ab libraries via simple, fast and inexpensive methods. In this regard, the universal QD-SpA platform features on-demand, flexible, single-step, purification-free QD-Ab assembly, along with high probe specificity (as intact Abs supplied in a variety of carrier buffers can be utilized). Further addressing requirements of the M3P technology, we have demonstrated that the SpA–Ab bond is sufficiently stable to avoid QD-SpA-Ab probe crosstalk. Previous works on decorating QD surface with various adaptor proteins are mainly based on highly charged species (QDs are often highly negatively charged [46] , [47] , [48] , [49] , whereas avidin and genetically engineered protein G are highly positively charged [46] , [47] , [49] ). Such probes have been used with some success for immunoassays and live-cell imaging, but exhibit extremely high nonspecific binding to fixed cells and tissue specimens, which limits their utility for highly multiplexed molecular profiling technology, especially when multiple cycles are utilized and substantial build-up of nonspecific signal becomes an issue. To avoid this problem, we used QDs coated with a non-fouling layer of PEG, which resists nonspecific binding even after bioconjugation with SpA and Ab. With this probe design, fully assembled functional QD-SpA-Ab allows direct target labelling for improved correlation between target expression and QD fluorescence signal, while the high brightness of QD probes makes imaging without signal amplification possible. Unique features of the novel QD-SpA nanoprobe provide a strong foundation for implementation of M3P technology. Besides offering a straightforward approach to preparation of an extensive customized QD-Ab library, dual use of intermediate SpA–Ab bond stability (i) prevents probe crosstalk during parallel multiplexed staining, while (ii) enabling quick probe dissociation and elution during specimen regeneration. As a result, several cycles of multicolour staining can be performed with a range of spectrally distinguishable QD probes on same specimens. In general, N colour staining performed for M cycles allows N × M molecular targets being probed. We have demonstrated the functionality of our QD-SpA-Ab probes using five targets as a model system. Yet, at this time, ten colours of spectrally distinguishable QDs are commercially available, which is coincident with the current colour deconvolution capability of HSI. Preparation of QDs with narrower emission peaks and improvements in HSI could further increase the multiplexing capability of parallel staining beyond ten. Indeed, recent work on QD bandgap engineering has produced particles with emission profile as narrow as 14 nm (full width at half maximum or FWHM) [50] , in contrast to the particles used here with typical 25–30 nm FWHM. To break the limitations of parallel multiplexing, multicycle staining, implemented as part of M3P technology, increases the multiplexing power by another magnitude. In this work, we have demonstrated that at least ten staining cycles can be performed without loss of specimen antigenicity and cell morphology. Brief treatment with regeneration buffer leads to effective removal of QD–SpA–Ab complex and thus completely regenerates specimens for next-cycle staining, enabling re-staining of the same or probing of a different panel of molecular targets. In conclusion, we have developed a technically straightforward, yet analytically powerful, imaging platform for comprehensive in situ single-cell molecular profiling. Overcoming the fundamental limitations of conventional and nanoparticle-based methods, the functionality of our technology comes from the unique combination of favourable optical properties of QDs, flexible QD-Ab probe preparation and the ability to perform multiple cycles of staining/de-staining without affecting specimen antigenicity and cell morphology. We envision that further development of M3P technology, especially by integrating it with automated staining–imaging instruments, will offer exciting opportunities in systems biology, signalling pathway analysis, gene expression studies, molecular diagnostics and drug discovery. Synthesis and characterization of QD–SpA bioconjugates Amine-functionalized PEG-coated QDs (Qdot ITK amino (PEG) QDs, Invitrogen) with emission peaks centred at 525, 545, 565, 585 and 605 nm were used for the preparation of QD-SpA. QDs were activated with bifunctional crosslinker BS3 ( bis (sulfosuccinimidyl) suberate, Thermo Scientific), followed by covalent conjugation with SpA (Protein A from Staphylococcus aureus , Sigma-Aldrich). Hundred microlitre 2 μM QD solution in PBS was mixed with 1,000 molar excess of BS3 and incubated for 30 min at room temperature. Excess crosslinker was removed with NAP-5 column (GE Healthcare) pre-equilibrated with PBS. Handheld UV lamp was used to aid in the collection of activated QDs. Eluted QDs were concentrated down to 50 μl with 100 kDa MWCO concentrator (GE Healthcare), and 100 μl of 100 μM SpA solution in PBS was added. The reaction was incubated overnight at room temperature and purified by ultrafiltration for at least six times with Amicon Ultra 100 kDa MWCO centrifugal filter (Millipore). Purified QD-SpA probes were stored in PBS solution at 4 ° C. A UV-2450 spectrophotometer (Shimadzu) was used to measure QD light absorption and calculate concentration of QD-SpA probes. Hydrodynamic size (diameter) of PEG-coated and SpA-functionalized QDs was measured with Nano-ZS nanoparticle zetasizer (Malvern Instruments). Cell culture and processing HeLa cells (ATCC) were grown in glass-bottom 24-well plates (Greiner Bio-One) for 2–3 days to a density of ~80–90%. Humidified atmosphere at 37 °C with 5% CO 2 was maintained. MEM culture medium with L -glutamine (Invitrogen) supplemented with 10% fetal bovine serum (PAA Laboratories) and antibiotics (60 μg ml −1 streptomycin and 60 U ml −1 penicillin) was used. For IF staining procedure, cells were rinsed with tris-buffered saline (TBS), fixed with 4% formaldehyde in TBS for 20 min, permeabilized with 2% DTAC/TBS (dodecyltrimethylammonium chloride, Sigma-Aldrich) for 20 min followed by 0.25% TritonX-100/TBS for 5 min and washed five times with TBS. Fixed cells were stored in TBS at 4 °C. Imaging and signal analysis IX-71 inverted fluorescence microscope (Olympus) equipped with a true-colour charge-coupled device (QColor5, Olympus) and a HSI camera (Nuance, 420–720 nm spectral range, CRI, now Advanced Molecular Vision) was used for cell imaging. Low-magnification images were obtained with X20 dry objective (NA 0.75, Olympus) and high-magnification with X100 oil-immersion objective (NA 1.40, Olympus). Wide UV filter cube (330–385 nm band-pass excitation, 420 nm long-pass emission, Olympus) was used for imaging of all QD probes, while Yellow set cube (540–580 nm band-pass excitation, 610 nm long-pass emission, Chroma) was used for Alexa Fluor 568 detection. All images were acquired with cells attached to the coverslip bottom of the well and immersed in TBS without use of anti-fading reagents. Nuance image analysis software was used to unmix the obtained images based on the reference spectra of each QD component along with an extra channel for background fluorescence. In a false-colour composite image, brightness and contrast of each channel was automatically adjusted for best visual representation and clear depiction of relative target distribution, unless noted otherwise. For sequential staining, a permanent reference point was marked on the bottom of the well to aid in finding the same cell subset for each imaging cycle. Minor misalignment between different frames was adjusted manually, and the frames were merged into a false-colour composite image in Photoshop (Adobe Systems). For quantitative analysis, Nuance image analysis software was used to automatically identify regions of interest that included QD staining and excluded ‘blank’ non-stained areas within each QD channel. An average signal intensity throughout all regions of interest within a single image was recorded for each QD channel. Identical analysis was performed on 3–5 low-magnification images (containing at least 400 cells per field of view) taken from different fields of view of the same specimen to obtain an overall average cell staining intensity and assess variability of signal intensity throughout the specimen. Differential brightness of QD probes was quantified using bulk fluorescence measurement of QD solutions with HSI as well as reference singleplex staining of same targets with all QD colours. Appropriate correction factors were then applied during analysis to compensate for differential QD brightness. Two-step single-colour IF Monoclonal rabbit antibodies raised against Ki-67 (Epitomics) and Cox4 (Cell Signalling Technology), polyclonal rabbit Abs against Lamin A (Sigma Aldrich) and β-tubulin (Epitomics), and monoclonal mouse anti-HSP90 Ab (IgG2a sub-type, Thermo Scientific) were used for technology validation. All buffers were prepared with deionized water (>18 MΩ cm). Blocking buffer composition was 2% BSA (from bovine serum albumin powder, Sigma-Aldrich), 0.1% casein (from 5% solution, Novagen), and 1 × TBS. Staining buffer composition was 6% BSA in 1 × TBS. Staining was performed with either dye-labelled secondary antibodies (rabbit-anti-mouse and goat-anti-rabbit IgG, Sigma-Aldrich, labelled with Alexa Fluor 568 carboxylic acid succinimidyl ester, Invitrogen), QDs functionalized with secondary Ab fragments (Qdot goat F(ab′)2 anti-mouse or anti-rabbit IgG conjugates (H+L), Invitrogen) or QD-SpA probes prepared as described above. All staining steps were performed directly inside the wells of glass-bottom 24-well plate at ambient conditions. For a two-step IF, cells were blocked with blocking buffer for 1 h and incubated with 300 μl 1 μg ml −1 primary antibodies in staining buffer for 1.5 h. Then, cells were washed three times with TBS and incubated with either 300 μl 4 μg ml −1 dye-labelled 2′Ab, 5 nM QD-2′Ab or 20 nM QD-SpA in staining buffer for 1.5–2 h in the dark. Extra fluorescent labels were removed by rinsing cells with 1% BSA/0.1% casein/TBS twice and washing with TBS three times. Fluorescence imaging was done immediately following staining, unless stated otherwise. Multiplexed single-step IF Multiplexed IF studies were performed in parallel, sequential or combined parallel/sequential manner. Regardless of the staining type, cells were blocked with blocking buffer for 1 h as described in the two-step IF section. Concurrently, QD-SpA-Ab probes were prepared by incubating 6 μl 1 μM QD-SpA with 1.5 μl 0.2 mg ml −1 1′Ab for 1 h at room temperature. Each QD-SpA-Ab probe was prepared in a separate microcentrifuge tube. For parallel multiplexed staining, all probes were combined in a single tube, diluted to 300 μl with staining buffer and immediately applied to the pre-blocked cells. After 2 h staining, cells were rinsed with 1% BSA/0.1% casein/TBS twice and washed with TBS three times. Imaging was done immediately following staining. For single-colour sequential staining QD-SpA-Ab probes were prepared using the same QD-SpA incubated with different antibodies in separate microcentrifuge tubes. Then each probe was used for a single-step single-colour staining and imaging. Each staining cycle consisted of (i) pre-blocking, (ii) staining, (iii) imaging and (iv) de-staining. First three steps were identical to those for parallel staining. De-staining was performed by washing stained cells with 1 ml of regeneration buffer (composed of pH2.8 IgG elution buffer (Thermo Scientific) and 0.5% SDS (Sigma Aldrich)) three times for 5 min each. Following de-staining, cells were rinsed with TBS, washed twice with blocking buffer for 5 min each and blocked for 60 min (as part of next staining cycle). Combined parallel/sequential staining utilized a cocktail of multiple QD-SpA-Ab probes on each cycle (taking about 4 h to complete one cycle). QD-Ab probe crosstalk and interference studies Probe crosstalk and interference studies were performed in the same manner as parallel dual-colour staining described above, except that one QD–SpA conjugate was incubated with 1′Ab, while the other one was not. Following QD-SpA-Ab probe assembly, QD 1 -SpA-Ab and QD 2 -SpA were combined in a microcentrifuge tube, diluted to 300 μl in staining buffer and added to the pre-blocked cells. As a reference, to demonstrate the capability of QD-SpA probes to efficiently compete for 1′Ab in solution, both QD-SpA probes were mixed with 1′Ab in 300 μl of staining buffer and immediately applied to cells. After 2-h staining, cells were washed and imaged. HSI was used to unmix and quantitatively compare individual QD signals. QD545 and QD585 were used for this study. Intensity of the dimmer QD545 channel was scaled up two times compared with brighter QD585 channel to correct for differential brightness of QD probes. For quantitative analysis, correction factor of 1.7 was applied to QD545 signal to normalize it against QD585. Crosstalk effect was evaluated by the contribution of each QD to a total measured fluorescent signal. Interference effect was evaluated by comparing staining intensity produced by each QD 1 -SpA-Ab probe in the presence of competitor QD 2 -SpA relative to staining intensity produced by QD 1 -SpA-Ab probe alone. Specimen degradation studies HeLa cells grown in different wells of the same 24-well plate were subjected to 0–10 regeneration cycles and stained for either Lamin A or HSP90. Regeneration cycle consisted of the following steps: washing with TBS for 15 min, de-staining with regeneration buffer for 15 min, blocking with 2% BSA/0.1% casein/TBS for 30 min and incubating with staining buffer for 30 min. All cells were stained and imaged at the same time (as a result, for example, exposure to one regeneration cycle implied incubation in TBS for nine cycles before treatment with regeneration conditions). Cells were stained using a two-step procedure: first incubated with target-specific 1′Ab for 1.5 h, then washed with TBS and incubated with species-matched QD565-2′Ab for 1.5 h. For all cells, four distinct areas were imaged at low magnification using HSI camera, and average staining intensity was assessed. Exposure time and other imaging conditions were kept constant for all images taken to enable direct quantitative comparison of signal intensity. SPR analysis of SpA–IgG bond stability SPR measurements of SpA–IgG bond stability were carried out on Biacore T100 instrument (GE Healthcare). SpA was covalently immobilized on CM5 sensor chip. All studies were done in 150 mM NaCl, 10 mM HEPES pH 7.4 running buffer under continuous flow at 10 μl min −1 . Surface regeneration was performed with 10 mM glycine-HCl pH2 buffer. For binding/dissociation studies, rabbit anti-mouse IgG at 100 and 10 nM concentration was injected over SpA-modified and control surfaces. For 100 nM analyte concentration, binding was monitored for 10 min and dissociation for 30 min, while for 10 nM analyte concentration times were 30 and 60 min, respectively. During dissociation step, surface was continuously washed with running buffer. The data analysis was carried out using the BIAevaluation 2.0 software. How to cite this article: Zrazhevskiy, P. and Gao, X. Quantum dot imaging platform for single-cell molecular profiling. Nat. Commun. 4:1619 doi: 10.1038/ncomms2635 (2013).